Warming and nitrogen deposition lessen microbial residue contribution to soil carbon pool Microorganisms have a role as gatekeepers for terrestrial carbon fluxes, either causing its release to the atmosphere through their decomposition activities or preventing its release by stabilizing the carbon in a form that cannot be easily decomposed. Although research has focused on microbial sources of greenhouse gas production, somewhat limited attention has been paid to the microbial role in carbon sequestration. However, increasing numbers of reports indicate the importance of incorporating microbial-derived carbon into soil stable carbon pools. Here we investigate microbial residues in a California annual grassland after a continuous 9-year manipulation of three environmental factors (elevated CO 2 , warming and nitrogen deposition), singly and in combination. Our results indicate that warming and nitrogen deposition can both alter the fraction of carbon derived from microbes in soils, though for two very different reasons. A reduction in microbial carbon contribution to stable carbon pools may have implications for our predictions of global change impacts on soil stored carbon. Studies of soil organic carbon (C) dynamics have markedly increased in number due to growing interest in understanding the global C cycle as it pertains to climate change [1] , [2] , [3] . As soil C cycling is ultimately a consequence of microbial growth and activity, the mechanistic basis for C decomposition, transformation and stabilization in soils depends on a detailed understanding of microbial physiology and activities. Although it is readily accepted that soil C dynamics are heavily influenced by catabolic and anabolic activities of microorganisms [4] , [5] , the incorporation of microbial biomass components into soil stable C pools (via microbial living cells and necromass) has received less attention [6] . Nevertheless, reports indicate that senesced microbial biomass may have a far greater role in the stabilization of C into soil pools than traditionally believed [5] , [6] , [7] , [8] , [9] , [10] , [11] . General concerns about climate change have led to growing interest in the response of terrestrial ecosystems to multiple environmental changes. To date, the majority of studies on ecosystem C storage response triggered by climate change have been focused on the role of above-ground tissue chemistry and biomass production [12] , the dynamics of total terrestrial C capacity [13] , and more recently in identifying microbial indices of C utilization and activity that lead to trace gas production [14] , [15] , [16] , [17] . However, little is known about the degree to which soil microbial-derived C persists in the soil, and contributes to stable C. Microbial production of recalcitrant organic C lies at the root of two issues of global concern—maintaining soil productivity and controlling greenhouse gas levels [7] . Studies focused on microorganisms and stable C will help increase our understanding of global biogeochemical cycles and advance the current state of knowledge of global C cycle models [7] , [18] . To predict future changes in microbial-derived C and its response to disturbance it is essential we understand the intrinsic mechanisms underlying its persistence and transformation. In particular, there is a need for studies that address whether environmental change drivers will accelerate or slow the accumulation of microbial-derived C in soil. Direct measurement of C from microbial residues is difficult as differentiation between the C bound in microbial residues and that in background soil organic C is technically very difficult. Alternatively, studies of microbial biomarker amino sugars can be used as a time-integrated measure of the contribution of dead microbial cells to soil organic C pools [19] , [20] , [21] , [22] . In this study, we quantified the microbial amino sugars in surface soils from a California annual grassland ecosystem after a 9-year manipulation of three global change factors at the Jasper Ridge Global Change Experiment (JRGCE) [23] . Our goal was to investigate the impact of multiple interacting global change drivers on microbial residue production and soil C dynamics. Our results show that warming and nitrogen (N) deposition can both alter the fraction of C derived from microbes in soils. Dynamics of soil microbial residue abundance in JRGCE We quantify microbial amino sugars in surface soils (0–10 cm) from a California annual grassland ecosystem after a continuous 9-year manipulation of three global change factors (elevated CO 2 , warming and N deposition), alone or in combination, at the JRGCE [23] . We report microbial residue abundance using amino sugar proportion of soil total C (AS/TC), indicating relative accumulation of microbial residues in the soil C pool. At the Jasper Ridge grassland experiment, we found that CO 2 was not a direct factor influencing soil amino sugar and total C pools, and that the amino sugar fraction of the soil total C pool (the AS/TC ratio) was unaffected by elevated CO 2 . In contrast, the AS/TC ratio significantly declined after exposure to increased temperature and elevated N levels ( Fig. 1 ). Both warming and N deposition showed a significant decrease in the fraction of C derived from microbes in soils. In both cases, we observed a significantly lower soil AS/TC ratio, though for two different reasons. Under warming, amino sugars decreased substantially and soil total C remained relatively constant, whereas under N deposition total soil C increased and amino sugars decreased slightly ( Fig. 1 ). It is thus likely that two different mechanisms explain the lowered soil AS/TC ratio. 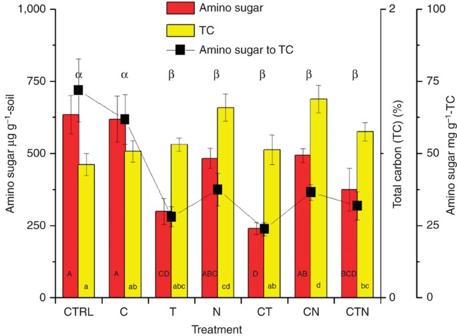Figure 1: Total carbon and amino sugar abundances in JRGCE. The effect of single and combined global environmental change treatments on the total C pool, amino sugar pool and the proportion of amino sugars in the total C pool. Error bars indicate s.e.m. (n=4 or 5). Treatments sharing a letter are not significantly different (P<0.05, multiple comparison test by least significant difference). The greek alphabets denote significance for the ratio of amino sugars to total C, the capital letters for amino sugars and lowercase letters for total C. CTRL, control; C, elevated CO2; T, elevated temperature; N, nitrogen deposition. Figure 1: Total carbon and amino sugar abundances in JRGCE. The effect of single and combined global environmental change treatments on the total C pool, amino sugar pool and the proportion of amino sugars in the total C pool. Error bars indicate s.e.m. ( n =4 or 5). Treatments sharing a letter are not significantly different ( P <0.05, multiple comparison test by least significant difference). The greek alphabets denote significance for the ratio of amino sugars to total C, the capital letters for amino sugars and lowercase letters for total C. CTRL, control; C, elevated CO 2 ; T, elevated temperature; N, nitrogen deposition. Full size image Warming appeared to decrease microbial contribution to stable C substantially while having minimal impact on total soil C levels. The reduction in microbial contribution is possibly due to preferential degradation of amino sugars under warmer soil conditions [24] . However, it is more likely due to a decline in growth or increase in turnover rate either due to heat stress or a shift in community composition to organism with lower biomass production. The literature indicates that microorganisms subject to heat stress may respond by decreasing their overall biomass [15] or decreasing the fraction of assimilated C that is allocated to their growth [25] . In the case of N addition, in contrast, total soil C increased, whereas microbial amino sugars decreased slightly. The net result was an overall decline in the AS/TC ratio similar to that under warming but for a different reason. The JRGCE grassland is N-limited, and plant biomass responds positively to added N (ref. 26 ). In addition, when nutrient limitation is relieved, we see a distinct decline in arbuscular mycorrhizal fungi abundance in these soils [17] . It is likely that this decline in arbuscular mycorrhizal fungi is driving the overall decline in microbial contribution to total soil C. Admittedly, these data are drawn from a single measure in time, in a single study. However, they represent a 9-year exposure to continuous environmental manipulation. In addition, amino sugars are a robust integrative measure of microbial C, not subject to rapid fluctuations [20] , [21] , [27] . We feel that the occurrence of these two distinct potential mechanisms regulating microbial production of soil C underscores the importance of looking beyond simple or single measures of microbial community, biomass or soil C. The mechanism that drives change in stable soil C may not be obvious. In this study, the use of microbial residue biomarker analysis allows us to distinguish soil C of direct microbial origin from other fractions [10] . Microbial amino sugars are relatively recalcitrant, and represent part of the soil stable C pool. The soil stable C pool has a critical role as a C sink within the global C cycle, and even a small change in this pool could have large consequences for atmospheric chemistry when other pools do not change to compensate. The sensitivity of microbial residues to warming and N deposition observed in this study therefore may have implications for our predictions of global change impact on soil C. The ‘microbial carbon pump’, a recently proposed conceptual framework, has been highlighted for understanding the role of microbes in production of recalcitrant organic C and C storage in the ocean [18] , [28] , [29] . We propose that a similar ‘pump’ operates in the soil [7] , [18] . The reduction in microbial C contribution to soil C pool observed in this study may indicate a malfunction of the microbial carbon pump in soil under warming and N deposition, and the potential consequences may be severe—stable soil C accumulates and forms over hundreds and thousands of years, yet can be lost very quickly. It may be difficult if not impossible to recover or restore this C on decadal timescales, and change in soil C cycling may substantially disrupt the C source-sink balance of terrestrial systems under global climate change. Jasper Ridge Global Change Experiment The JRGCE was established in a grassland ecosystem in the eastern foothills of the Santa Cruz Mountains at the Jasper Ridge Biological Preserve in the San Francisco Bay area [23] . The region experiences a Mediterranean climate, and is generally dominated by annual non-native grasses Avena barbata and Avena fatua . The experiment was initiated in fall of 1998 with a randomized block design, containing continuous manipulations of each of the following global change factors with two levels: atmospheric CO 2 concentration (350 and 700 ppm), temperature (+1°C at the soil surface and a no heat control), N addition (ambient and 7 g Nm −2 per year). Our analysed soils were sampled in April of 2007, corresponding with peak plant growth. Total soil C and N data were determined by combustion analysis and provided by the JRGCE facility support staff. Amino sugar analysis The amino sugar analysis method was adapted from a previous protocol [30] , [31] , as modified by Liang et al . [32] Briefly, ~1 g lyophilized soil samples were heated for 8 h at 105 °C in closed hydrolysis flasks with 6 M HCl. The hydrolysate was dried completely by rotary evaporation at 40 °C under partial vacuum, taken up into methanol, transferred to 3-ml vials and evaporated to dryness on a Labconco 79000 RapidVap (Labconco Co., Kansas City, MO, USA). The residues were re-dissolved in 1 ml distilled deionized H 2 O, lyophilized overnight and then processed for aldononitrile acetate derivatization. To prepare the aldononitrile derivatives, the amino sugars were dissolved in a derivatization reagent consisting of hydroxylamine hydrochloride (32 mg ml −1 ) and 4-(dimethylamino) pyridine (40 mg ml −1 ) in 4:1 (v/v) pyridine-methanol, and heated to 75–80 °C for 35 min. Then, 1 ml acetic anhydride was added, and the solution was reheated for 25 min for acetylation. After cooling, 1.5 ml dichloromethane and 1 ml HCl were successively added and the mixture was vortexed to transfer the amino sugars to the organic phase. The solution was washed thrice with 1 ml deionized H 2 O to remove excess derivatization reagents. In the last washing step, the aqueous phase was removed as completely as possible. Finally, the organic phase was dried at 45 °C in a Labconco 79000 RapidVap (Labconco Co) and resuspended in 300 μl ethyl acetate-hexane (1:1) for gas chromatography. Gas chromatography-flame ionization detection analysis of the aldononitrile acetate derivatives was conducted on an Agilent model 6890 GC (Wilmington, DE, USA) equipped with a split/splitless inlet and flame ionization detection. Sample extracts (2 μl) were injected onto a J&W Scientific Ultra-2 column (25 m × 0.2 mm × 0.33 μm) using H 2 as the carrier gas at a constant flow rate of 0.4 ml min −1 . The GC inlet was set to 250 °C and operated in split mode with a 30:1 ratio. Myo-inositol (internal standard) and N -methylglucamine (recovery standard) were used as standards. Derivatives of each pure amino sugar standard were prepared in an identical manner for calibrating response factors to the internal standard. Sum of individual amino sugars were applied to represent soil amino sugar pool. How to cite this article: Liang, C. & Balser, T.C. Warming and nitrogen deposition lessen microbial residue contribution to soil carbon pool. Nat. Commun. 3:1222 doi: 10.1038/ncomms2224 (2012).